Camelid genomes reveal evolution and adaptation to desert environments Bactrian camel ( Camelus bactrianus ), dromedary ( Camelus dromedarius ) and alpaca ( Vicugna pacos ) are economically important livestock. Although the Bactrian camel and dromedary are large, typically arid-desert-adapted mammals, alpacas are adapted to plateaus. Here we present high-quality genome sequences of these three species. Our analysis reveals the demographic history of these species since the Tortonian Stage of the Miocene and uncovers a striking correlation between large fluctuations in population size and geological time boundaries. Comparative genomic analysis reveals complex features related to desert adaptations, including fat and water metabolism, stress responses to heat, aridity, intense ultraviolet radiation and choking dust. Transcriptomic analysis of Bactrian camels further reveals unique osmoregulation, osmoprotection and compensatory mechanisms for water reservation underpinned by high blood glucose levels. We hypothesize that these physiological mechanisms represent kidney evolutionary adaptations to the desert environment. This study advances our understanding of camelid evolution and the adaptation of camels to arid-desert environments. The evolution and adaptation of desert animals to their environment at the genome level remains largely unknown. Camels ( Camelus , Camelini) contain two extant domesticated species: the two-humped Bactrian camel and single-humped dromedary. These species live in the extreme desert environments of Africa and Asia, and their adaptations to arid conditions include a tolerance of temperatures exceeding 40 °C and water losses greater than 25% of total body weight [1] (in non-desert mammals, losses of greater than 15% are fatal [2] ). In contrast, their nearest relatives (Lamini), which have no hump and consist of two wild species (guanaco and vicuña) and two domesticated species (llama and alpaca), live in the high altitudes of South America and do not exhibit similar adaptations to hot desert environments ( Supplementary Fig. 1 ). The Bactrian camel, dromedary, llama and alpaca are important not only as beasts of burden for transport but also as sources of meat, milk and wool. In addition, both the dromedary and Bactrian camel represent ideal models for studying desert adaptation among mammals. Genomic research into the evolutionary history of camelid species and the unusual adaptations of camels to arid-desert environments has been limited, although recent studies have focused on the divergence time between the ancestors of the Bactrian camel and cattle, genomic single-nucleotide polymorphism (SNP) rates, population parameters, artificial domestication, insulin resistance, salt tolerance and other factors [3] , [4] . In this study we perform high-quality whole-genome sequencing of the Bactrian camel, dromedary and alpaca, and transcriptome sequencing of the Bactrian camel. Our results reveal the divergence times and demographic history of these species. These genomic and transcriptomic analyses provide evidence of camel adaptation to desert environments. Our analysis also provides numerous insights into the unusual physiological features and genetic architecture that enable camels to survive in desert environments. Genome sequencing and assembly We sequenced the genomes of a female Bactrian camel (79.3-fold coverage), a male dromedary (65.0-fold coverage) and a female alpaca (72.5-fold coverage) using the Illumina HiSeq2000 platform. The present estimated genome size of the Bactrian camel (2.45 Gb) is comparable with that of a previous report (2.38 Gb) based on K-mer analysis [3] . The assembled genome sizes for the three individuals were 2.01, 2.01 and 2.05 Gb, respectively ( Supplementary Tables 1–10 and Supplementary Figs 2 and 3 ). The present assembled genome size for the Bactrian camel is identical to the previously reported size [3] . 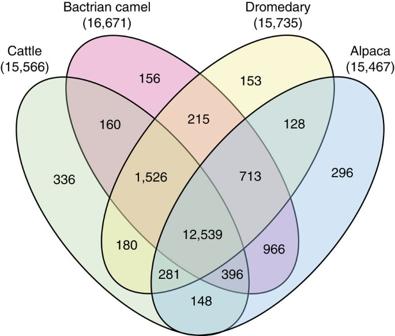Figure 1: Unique and homologous gene families. The number of unique and shared gene families is shown in each of the diagram components and the total number of gene families for each animal is given in parentheses. The contig N50 and scaffold N50 lengths ( Table 1 ) were 24.9 kb and 8.7 Mb for the Bactrian camel, 54.1 kb and 4.1 Mb for the dromedary, and 66.3 kb and 5.1 Mb for the alpaca, respectively. Compared with the genome of the wild Bactrian camel [3] , the present genomes of these three camelids have shorter contig N50 lengths but larger scaffold N50 lengths. Mapping of libraries with an insert size of 2 kb to the scaffold indicated that each of the genome sequences was of high quality ( Supplementary Fig. 4 and Supplementary Methods ), and the Bactrian camel transcriptome also demonstrated a high-quality genome assembly for the present and wild Bactrian camel [3] ( Supplementary Tables 11 and 12 ). The camelid genomes shared high synteny with the human and cattle reference genomes (coverage rate >83%) and a relatively low rate of genomic rearrangement within the Camelidae ( Supplementary Tables 13 and 14 , and Supplementary Methods ). The synteny between the Bactrian camel and cattle genomes observed in the present study is greater than that reported previously [3] . Our study supports the notion that divergent evolution in Camelidae occurred through single gene mutations or minor chromosomal rearrangements [5] . We estimated the segmental duplication of these three individuals: the total length of segmental duplication in both the Bactrian camel and dromedary was 26 Mb, smaller than that of the alpaca (36 Mb) ( Supplementary Table 15 ). The segmental duplication among these three organisms is lower than that reported in cattle (94.4 Mb) [6] . Table 1 Genomes statistics for three camelids. Full size table Genome annotation Using a combination of homologous sequence searches and ab initio gene predictions, we annotated 20,251, 20,714 and 20,864 genes in the Bactrian camel, dromedary and alpaca genomes, respectively ( Supplementary Fig. 5 , and Supplementary Tables 16 and 17 ). We used the CEGMA method [7] , which includes 458 core eukaryotic genes, to assess the completeness of the genomes and annotation. The vast majority of these core genes were aligned to the camelid genomes (99.12% for Bactrian camel, 98.47% for dromedary and 99.12% for alpaca), and the majority were present in our predicted gene sets (97.82% for Bactrian camel, 96.73% for dromedary and 93.87% for alpaca), supporting the completeness of the assembled genomes and gene sets identification ( Supplementary Tables 18–20 ). Comparative analyses of the three camelid gene sets revealed a high gene sequence similarity (>90%) but different non-synonymous/synonymous ( Ka / Ks ) distributions ( Supplementary Figs 6 and 7 ). Functional analyses of the gene sets indicated that >91% of the genes were functionally annotated in each genome ( Supplementary Tables 21–23 ). The repeat sequence content of the camelid genomes (30.4% in Bactrian camel, 32.1% in alpaca and 28.4% in dromedary) was 10% lower than that of cattle (42.5%) and humans (46.1%) due to the small number of short interspersed nucleotide elements in the camelid genomes ( Supplementary Tables 24–27 ). The repeat sequence content of the Bactrian camel genome was similar to that reported previously [3] . Annotation of non-coding RNA genes revealed similar copy numbers for each genome (Bactrian camel=1,942; dromedary=2,209; alpaca=2,328; Supplementary Tables 28–30 ). We identified 12,539 homologous gene families that are shared by 4 species in the order Cetartiodactyla (Bactrian camel, dromedary, alpaca and cattle): 156, 153 and 296 gene families were specific to the Bactrian camel, dromedary and alpaca, respectively ( Fig. 1 ). Figure 1: Unique and homologous gene families. The number of unique and shared gene families is shown in each of the diagram components and the total number of gene families for each animal is given in parentheses. Full size image Evolutionary analysis and phylogeny A phylogenetic tree was constructed including the camelids (Bactrian camel, dromedary and alpaca) and seven other species (cattle, horse, dog, panda, human, mouse and opossum). The tree was generated using PhyML [8] based on fourfold degenerate codon sites extracted from 7,398 single-copy orthologous genes identified by TreeFam [9] ( Supplementary Table 31 , and Supplementary Figs 8 and 9 ). 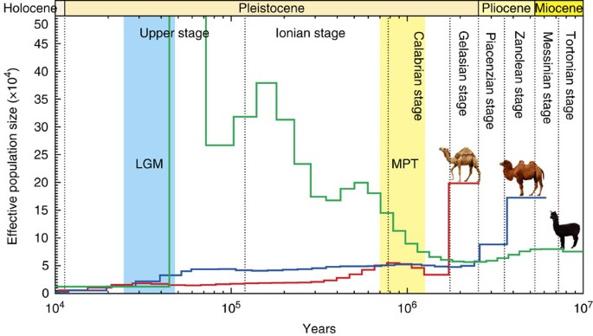Figure 3: Demographic history. The blue, red and green line represent the estimated population size of Bactrian camel, dromedary and alpaca, respectively. The geological time boundaries15of each unit from the Miocene Epoch to the Holocene Epoch are marked using broken lines. The middle Pleistocene transition (MPT) is highlighted in orange, while the Last Glacial Maximum (LGM) of South America is highlighted in blue. The estimated divergence time between camelids and cattle is 42.7 million years ago (Mya) ( Fig. 2 and Supplementary Fig. 10 ). This result is consistent with the time (45.9 Mya) at which palaeontological evidence indicates that the Camelidae family first appeared in North America [10] but is in contrasts with a previous estimate of the time of divergence of the cattle and Bactrian camel lineages based on 332 orthologues (55–60 Mya) [3] . The estimated divergence time of the ancestors of alpaca and the two camels (16.3 Mya) is consistent with palaeontological findings, indicating that the division between Camelini and Lamini occurred in North America ~17 Mya (ref. 10 ). The divergence time between the Bactrian camel and dromedary is ~4.4 Mya, implying they probably diverged after their common ancestor migrated from North America to Eurasia via the Bering Isthmus during the Late Miocene (7.246–4.9 Mya) [10] , [11] . We analysed the branch-specific Ka / Ks substitution ratios ( ω ) for these ten mammals using the method of Kosiol et al . [12] : the Bactrian camel and dromedary had higher branch ω -values ( Supplementary Fig. 11 , Supplementary Table 32 and Supplementary Methods ). 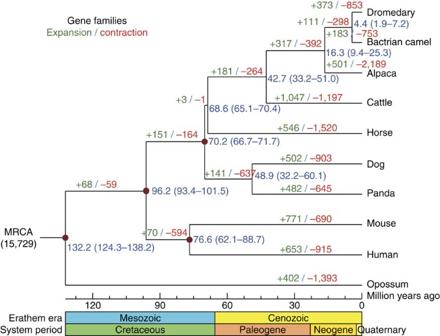This accelerated evolution in camels raises the possibility of camel-specific evolution to adapt to a desert environment. Figure 2: Phylogenomic analysis. The number of expanded (green) and contracted (red) gene families is shown at each branch. The red points on the four internal nodes indicate the fossil calibration times that were used in the analysis. The estimated divergence time (Mya) of each evolutionary lineage is shown in blue. The blue numbers in brackets are confidence intervals. MRCA, most recent common ancestor. Figure 2: Phylogenomic analysis. The number of expanded (green) and contracted (red) gene families is shown at each branch. The red points on the four internal nodes indicate the fossil calibration times that were used in the analysis. The estimated divergence time (Mya) of each evolutionary lineage is shown in blue. The blue numbers in brackets are confidence intervals. MRCA, most recent common ancestor. Full size image Heterozygote rates and demographic history SNPs were identified using SOAPsnp [13] . The estimated heterozygote rates of the Bactrian camel, dromedary and alpaca genomes were 1.16 × 10 −3 , 0.74 × 10 −3 and 2.66 × 10 −3 , respectively ( Supplementary Tables 33–35 ). The heterozygote rate of the Bactrian camel estimated here is comparable to that reported previously (1.0 × 10 −3 and 1.29 × 10 −3 ) [3] , [4] . The genomic SNP distributions among these mammals are different ( Supplementary Fig. 12 ). The demographic history of these camelids was constructed based on SNP data by applying the pair-wise sequentially Markovian coalescent (PSMC) model [14] ( Fig. 3 ). The results of our analysis indicated that the ancestor of the Bactrian camel had stable population sizes following two declines that occurred 3.69 and 2.61 Mya. Two declines in population size occurring 1.72 and 0.77 Mya were calculated for the ancestor of the dromedary. These estimated declines in the population size of the ancestors of both species are consistent with transitions between geological ages, including the Zanclean and Piacenzian (3.60 Mya), the Piacenzian and Gelasian (2.59 Mya), the Gelasian and Calabrian (1.81 Mya), and the Calabrian and Ionian (0.78 Mya) [15] , suggesting a probable correlation. Moreover, the expansion of the ancestral population of the dromedary occurred between 1.25 and 0.77 Mya, coinciding with the middle Pleistocene transition from 1.25 to 0.70 Mya, a period of fundamental changes in the Earth’s climatic cyclicity [16] that had a profound effect on the distribution and evolution of biota [17] . This time interval also coincides with the Galerian Mammal Age (1.2 to 0.60 Mya), which was characterized by a renewal of fauna that, in some cases, gave rise to new species that were adapted to arid, cold climates [18] ; more importantly, however, this time interval also coincides with the maximal diversity of the family Camelidae, which occurred in the early Galerian [19] . This correlation supports the adaptation of the ancestor of the dromedary to environmental changes and an expansion of its population during the middle Pleistocene transition. The most recent decrease in the population of the Bactrian camel ancestor occurred ~60 thousand years ago (Kya), which corresponds to the dispersal of modern humans out of Africa to Eurasia [20] , home of the Bactrian camel. Therefore, human activities may have impacted the recent ancestral population of the Bactrian camel. Figure 3: Demographic history. The blue, red and green line represent the estimated population size of Bactrian camel, dromedary and alpaca, respectively. The geological time boundaries [15] of each unit from the Miocene Epoch to the Holocene Epoch are marked using broken lines. The middle Pleistocene transition (MPT) is highlighted in orange, while the Last Glacial Maximum (LGM) of South America is highlighted in blue. Full size image The effective population size of the ancestor of the alpaca gradually decreased between ~5.37 Mya, which is closer to the time boundary of the Messinian and Zanclean stage (5.33 Mya) [15] , and 2.09 Mya, which is in the Uquian age (3 to 1.2 Mya), during which the ancestor of the alpaca migrated to South America through the Panamanian land bridge in the Great American Biotic Interchange [21] . This suggests that the migration may have contributed to the reduction in the population size of the ancestor of the alpaca. Its population size then expanded during the Pleistocene, followed by three periods of major bottlenecks before 501, 139 and 44 Kya. The population underwent a major expansion ~72 Kya, reaching a size of ~113 × 10 4 individuals. The most recent bottleneck (44 Kya) corresponds to the Last Glacial Maximum (48–25 Kya), which was advanced in South America [22] , and resulted in a dramatic reduction in population size to ~1.2 × 10 4 individuals. This implies that the cold conditions in South America at that time may have resulted in the constriction of the population size of the ancestor of the alpaca towards the end of the Pleistocene. Gene evolution We next investigated camelid genes that underlie adaptation to the environment. We adopted CAFÉ [23] to identify gene families that have undergone significant expansion and contraction during evolution ( Fig. 2 and Supplementary Methods ) and identified 373 expanded and 853 contracted gene families in the dromedary genome, 183 expanded and 753 contracted gene families in the Bactrian camel genome and 501 expanded and 2,189 contracted gene families in the alpaca genome. Many of the expanded gene families in these three camelids are significantly enriched in the cellular process, cell part, olfactory receptor activity, iron and immune-related Gene Ontology (GO) categories ( Supplementary Figs 13–15 and Supplementary Tables 36–38 ). We identified 287 positively selected genes (PSGs) in the Bactrian camel ( Supplementary Data 1 ), 324 PSGs in the dromedary ( Supplementary Data 2 ) and 151 PSGs that were common to both genomes, indicating similar selective pressures. An assessment of unique amino acid residue changes in orthologous genes that are present in 23 species identified 350 and 343 altered genes in the Bactrian camel and dromedary, respectively. Several overrepresented categories of genes with unique amino acid residue changes in camels were related to catalytic activity, small molecule binding and ATP binding ( Supplementary Figs 16 and 17 , and Supplementary Tables 39 and 40 ). Based on an analysis of syntenic blocks, 190 gained genes were identified in the Bactrian camel and 126 in the dromedary. These gained genes are significantly enriched in the olfaction and immune-related categories ( Supplementary Tables 41 and 42 , and Supplementary Methods ). Energy and fat metabolism As energy is important for camels living in food-scarce deserts, the selection of genes involved in energy-related processes was analysed. The genome-wide features of adaptation were identified by GO categories with lineage-specific accelerated evolution ( Supplementary Data 3–14 ). In contrast to cattle, the common rapidly evolving GO categories of the three camelids included cellular response to insulin stimulus (GO:0032869, P <0.001) and the insulin receptor signalling pathway (GO:0008286, P <0.001) ( Supplementary Data 4, 8 and 14 ). In addition, we identified a number of categories associated with energy, glucose and fat metabolism that evolved more rapidly in these camelids than in cattle. Some of the energy-related GO categories identified as evolving more rapidly in the Bactrian camel than in cattle are consistent with those reported previously [3] . Moreover, 13 genes involved in mitochondrial function, β-oxidation and cholesterol synthesis and transport had amino acid residue changes that were unique to the Bactrian camel and dromedary. Several genes ( ACC2 , DGKZ and GDPD4 ) involved in fat metabolism underwent expansion in the Bactrian camel genome, while the expanded gene families of the dromedary were enriched in the mitochondrion (GO:0005739, P =2.30 × 10 −5 ) category ( Supplementary Table 37 ). The different number of humps in these three camelids may reflect their distinct fat metabolism abilities. 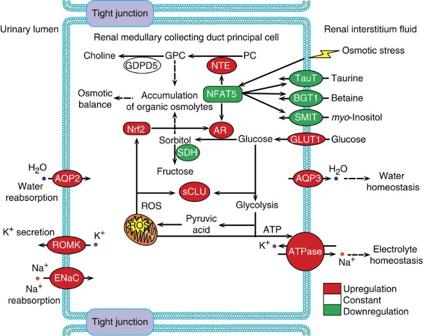Figure 4: Schematic model of renal medullary osmosis and water reservation in the camel under water restriction. The shading of boxes indicates the upregulation (red), constant expression (white) or downregulation (green) of genes in the renal medulla of Bactrian camels during WR. The dashed lines indicate the ultimate functions or effects of the gene expression and the related product’s activities. Functional categories associated with ATP (GO:0006200, GO:0016887, GO:0042626, P <0.01), mitochondria (GO:0005739, GO:0005759, P <0.01), lipid transport (GO:0006869, P Bactrian camel =5.33 × 10 −5 , P dromedary =0.00016) and response to insulin stimulus (GO:0032868, P Bactrian camel =0.0005, P dromedary =1.33 × 10 −5 ) evolved rapidly in both camel species compared with the alpaca ( Supplementary Table 43 ). Categories associated with lipid metabolism evolved more rapidly in the Bactrian camel than in the dromedary, for example, lipid catabolic process (GO:0016042, P =0.0015) and fat cell differentiation (GO:0045444, P =2.54 × 10 −9 ) ( Supplementary Table 44 ). These genes may enhance the energy storage and production capacity of a camel in the desert and may also reflect a difference in fat metabolism and in turn be related to the number of humps. Stress response To investigate adaptations to arid and hot environments, we further analysed genes involved in stress responses. Compared with cattle, categories associated with DNA damage and repair (GO:0006974, GO:0003684, GO:0006302, P< 0.01), apoptosis (GO:0006917, GO:0043066, P< 0.01), protein stabilization (GO:0050821, P Bactrian camel =0.00021, P dromedary =3.44 × 10 −19 ) and immune responses (GO:0006955, GO:0051607, P <0.01) exhibited accelerated evolution in both camel species ( Supplementary Data 8 and 14 ). Compared with the alpaca, significant functional categories were identified for T-cell co-stimulation (GO:0031295, P Bactrian camel =8.67 × 10 −32 , P dromedary =9.33 × 10 −9 ), oxidation–reduction processes (GO:0055114, P Bactrian camel =4.88 × 10 −15 , P dromedary =5.22 × 10 −21 ) and oxidoreductase activity (GO:0016491, P Bactrian camel =2.27 × 10 −10 , P dromedary =7.23 × 10 −7 ), all of which exhibited accelerated evolution in both camels ( Supplementary Data 6 and 12 ). Three genes ( ERP44 , NFE2L2 and MGST2 ) were correlated with oxidative stress responses and featured unique amino acid residue changes in both camel genomes. The expanded gene families of the dromedary were enriched in cytochrome c oxidase activity (GO:0004129, P =5.80 × 10 −10 ) and monooxygenase activity (GO:0004497, P =1.32 × 10 −5 ) ( Supplementary Table 37 ). These results provide evidence of selection in camels to adapt to the harsh arid conditions of the desert environment. Adaptation of the respiratory system Another challenge of the desert environment is airborne dust, which can lead to respiratory diseases such as asthma. Thirteen PSGs in both camels, including FOXP3 , CX3CR1 , CYSLTR2 and SEMA4A , were related to respiratory diseases in humans. We also found that the lung development GO category (GO:0030324, P Bactrian camel =3.26 × 10 −5 , P dromedary =1.18 × 10 −19 ) ( Supplementary Data 6 and 12 ) evolved rapidly in the dromedary and Bactrian camel compared with the alpaca. Selection of these genes provides further evidence of the adaptation of camels to endure the challenges of the desert environment. Adaptation of the visual system Solar radiation is another aspect of the desert environment. Long-term exposure to ultraviolet radiation can lead to a number of ophthalmic conditions. We examined genes that might accustom the eyes of camels to the extreme solar irradiation in the desert and identified positive selection at the OPN1SW , CX3CR1 and CNTFR genes, which are related to photoreception and visual protection, in both camels. The results also indicated that visual perception (GO:0007601, P Bactrian camel =0.0018, P dromedary =2.49 × 10 −14 ) evolved rapidly in both camels compared with the alpaca ( Supplementary Data 6 and 12 ). These results suggest a genetic basis for the ability of camels to endure prolonged exposure to ultraviolet light without damage to the visual system. Salt metabolism We then focused on the salt metabolism of camels by considering the main effect of salt on water balance. In contrast to a previous report on salt tolerance [3] , our results indicated that the category of sodium ion transport (GO:0006814, P Bactrian camel =0.0014, P dromedary =0.00012) evolved more rapidly in both camels than in cattle ( Supplementary Data 8 and 14 ). The category associated with the voltage-gated potassium channel complex (GO:0008076, P Bactrian camel =8.77 × 10 −8 , P dromedary =2.68 × 10 −10 ) evolved rapidly in both camels compared with the alpaca ( Supplementary Data 6 and 12 ). Notably, the genome of the Bactrian camel contains two copies of the NR3C2 and IRS1 genes, both of which play critical roles in sodium reabsorption and water balance in the kidney [24] , [25] , [26] , whereas other mammals possess only a single copy of each gene. This difference suggests that camels may metabolize and transport salt more efficiently than alpaca and cattle, and these pathways are important for water reabsorption. Differentially expressed genes and enrichment analysis To obtain greater insight into the characteristics of adaptation to the arid desert, we sequenced the renal cortical and medullary transcriptomes of a group of Bactrian camels after 24 days of water-restricted (WR) conditions and those of a control group (CG) ( Supplementary Table 45 , and Supplementary Data 15 and 16 ). We selected significantly upregulated or downregulated genes in these tissues ( Supplementary Figs 18–21 and Supplementary Methods ) and then analysed the enriched GO categories of these genes ( Supplementary Figs 22–25 , Supplementary Data 17–20 and Supplementary Methods ). An overrepresentation of categories associated with metal ion binding (GO:0046872, P =1.53 × 10 −23 ) and the regulation of body fluid levels (GO:0050878, P =1.37 × 10 −6 ) was detected in the set of upregulated renal cortical genes ( Supplementary Data 17 ). The GO categories associated with the glucose metabolic process (GO:0006006, P =4.11 × 10 −6 ), gluconeogenesis (GO:0006094, P =0.0026), mitochondrion (GO:0005739, P =2.13 × 10 −5 ), the generation of precursor metabolites and energy (GO:0006091, P =0.0077), response to nutrient levels (GO:0031667, P =0.0064) and response to stress (GO:0006950, P =0.0094) were enriched in the set of upregulated renal medullary genes ( Supplementary Data 19 ). Sodium reabsorption Genes encoding the Na + /K + -ATPase and the epithelial Na + channel (ENaC), which reabsorb sodium in the kidney, were upregulated in the renal cortex and medulla under WR conditions ( Supplementary Tables 46 and 47 ). The flexible transcription of the subunits of ENaC in different tissues and under different conditions suggests that the camel regulates the Na + reabsorbing activity of ENaC to cope with different physiological water requirements. These findings indicate that the regulation of sodium reabsorption may be essential for the survival of camels in a water-scarce environment. Water reservation The camel is renowned for its adaptation to prolonged water restriction. We therefore investigated the mechanism of water reservation by analysing the transcription of the aquaporin family genes, which are selective water channels with important functions in water reabsorption and metabolism. AQP1 , AQP2 and AQP3 were the top three differently expressed genes in the renal cortex and medulla under WR conditions ( Supplementary Tables 48 and 49 , and Supplementary Fig. 26 ). These genes may allow camels to reabsorb water more efficiently in a water-scarce environment. However, we did not detect AQP4 mRNA in the Bactrian camel kidney, consistent with its lack of expression in the desert rodent Dipodomys merriami merriami [27] but in contrast to its abundant expression in the human kidney [28] . Interestingly, a unique amino acid residue change (R261C) was observed in AQP4 in the Bactrian camel genome ( Supplementary Fig. 27 ). These findings may suggest a unique strategy for water reabsorption and metabolism in the camel kidney. Osmoregulation As hypertonicity is the foundation of water balance and reabsorption in the kidney, the expression of genes that are involved in osmoregulation in the renal medulla were analysed. Nuclear factor of activated T-cells 5 ( NFAT5 ), the only known tonicity-regulated transcription factor in mammals [29] , was expressed at 3.66% of the control level under WR conditions ( Supplementary Table 50 ). Accordingly, sodium/ myo -inositol cotransporter ( SMIT ), sodium- and chloride-dependent taurine transporter ( TauT ) and sodium- and chloride-dependent betaine transporter ( BGT1 ) exhibited reduced expression under WR conditions. These three transporters transactivated by NFAT5 transport compatible organic osmolytes into renal medullary cells (RMCs) in response to hypertonicity [30] ( Fig. 4 ). The downregulation of NFAT5 and its target genes during hypertonic stress has not been observed in other mammals [29] , [31] , including desert animals such as the Spinifex hopping mouse ( Notomys alexis ) [32] . Our findings indicate that camels may rely on other osmoregulatory strategies to protect against hypertonic stress during long-term water restriction. Figure 4: Schematic model of renal medullary osmosis and water reservation in the camel under water restriction. The shading of boxes indicates the upregulation (red), constant expression (white) or downregulation (green) of genes in the renal medulla of Bactrian camels during WR. The dashed lines indicate the ultimate functions or effects of the gene expression and the related product’s activities. Full size image Organic osmolytes The accumulation of organic osmolytes helps RMCs to balance the osmotic pressure between the intracellular and extracellular environments [30] . The downregulation of TauT , BGT1 and SMIT implies that the transport of taurine, betaine and myo -inositol into cells is decreased. Remarkably, we observed the transcriptional upregulation of aldose reductase ( AR ) and the downregulation of sorbitol dehydrogenase ( SDH ) in the sorbitol pathway; we also observed the transcriptional upregulation of neuropathy target esterase ( NTE ) and the stable transcription of glycerophosphodiester phosphodiesterase domain-containing protein 5 ( GDPD5 ) in the glycerophosphocholine (GPC) pathway ( Fig. 4 and Supplementary Table 50 ). The expression patterns of these genes suggest that in the camel, sorbitol and GPC may accumulate under WR conditions and that osmolytes may be mainly produced by the RMCs themselves. Sorbitol can serve as a source of energy [33] and help balance the osmolality of high extracellular NaCl [34] ; the energetic cost of the accumulation of GPC in response to high NaCl or urea in the renal medulla [30] may be less than that of transporting betaine into cells against a high concentration gradient [30] . Thus, these variations in the expression of osmolyte-related genes indicate that two osmolytes rather than five are principally used in response to hypertonicity as part of a low-energy-consumption model for camel survival in the food-scarce desert. Importantly, we observed that the expression levels of GLUT1 (glucose transporter 1) and genes involved in glycolysis were profoundly increased in the renal medulla under WR conditions ( Supplementary Table 51 ). Together with a previous report that the expression level of GLUT1 is induced by osmotic and metabolic stress [35] , our results suggest that the enhancement of glucose intake not only ensures a sufficient glucose concentration for the synthesis of sorbitol but also supplies the energy required for the upregulated Na/K-ATPase to maintain the internal ion gradient for adapted hypertonicity ( Fig. 4 ). Collectively, our observations suggest that the characteristic high blood glucose (6–8 mmol l −1 ) [36] , [37] of camels may be an adaptive evolutionary strategy for osmoregulation and water reabsorption of RMCs during antidiuresis. Osmoprotection Given the potential for hyperosmotic damage to cells [30] , we analysed the expression of genes related to cell protection and found that the expression levels of 25 genes encoding antioxidants and related enzymes ( Supplementary Table 52 ) were higher in the renal medulla under WR conditions. Genes encoding antioxidative transcription factors, including Nrf2, heat shock factor-1, activator protein-1 complex, p53, nuclear factor-κB and signal transducer and activator of transcription 4 also exhibited elevated expression in the WR renal medulla. In addition, we identified 14 heat shock genes, which contribute to the elimination of misfolded proteins under hyperosmolality [30] , that were upregulated in the WR renal medulla ( Supplementary Table 52 ). Gene clusterin , a cytoprotective chaperone, was dramatically increased by ~8.9-fold and had the highest transcription level in the WR renal medulla (reads per kilobase per million mapped reads=27,069). Previous studies have shown that clusterin is induced by glucose [38] and associated with diverse pathological states, including diabetes [39] and kidney injury [40] . The identification of clusterin as a PSG in the dromedary suggests that this gene may play a major role in the cytoprotection of the camel renal medulla during water restriction and that the high level of blood glucose in camels may serve a function during osmoprotection. Overall, the upregulation of osmoprotective genes indicates that camels have a sophisticated osmoprotective capability under WR conditions. Using deep sequencing and de novo assembly, we generated high-quality genome sequences of the Bactrian camel, dromedary and alpaca. Comparative genomic analyses provided new insights into the evolutionary history of these camelids and the adaptations of camels to the harsh desert environment. Transcriptome analyses revealed a network of genes that are involved in water reabsorption and glucose function in osmoregulation and water reservation, which suggests that the hyperglycemia that is characteristic of camels may be an adaptation to life in the water-scarce desert. The identification of key genes involved in the adaptation to the desert environment may have applications in breeding programmes and may provide some perspective for disease-resistance research. Future studies on camel genomes and transcriptomes may contribute to a detailed understanding of these important physiological mechanisms with relevance to human medical conditions (for example, the links between sodium metabolism and hypertension, hyperglycemia and diabetes, fat metabolism and obesity, and dust and respiratory diseases). Finally, in light of ongoing global warming and the increasing incidence of droughts, these camelid genomes are valuable resources for studying biological adaptations to environmental changes. Genome sequencing and assembly We used a whole-genome shotgun strategy and next-generation sequencing technologies on an Illumina HiSeq 2000 platform to sequence the genomes of a female Bactrian camel, a male dromedary and a female alpaca from blood DNA. A series of paired-end sequencing libraries with insert sizes of 170, 500 and 800 bp, and 2, 5 and 10 kb was constructed and sequenced for the Bactrian camel, dromedary and alpaca, respectively. An additional library with insert sizes of 20 kb was constructed for the Bactrian camel. The genomes of these three organisms were assembled using SOAP denovo (version 1.05) [41] . Gene prediction We used both homology-based and de novo methods to predict genes in the three genomes. For the homology-based prediction, gene sets from other species were mapped onto the genomes using TblastN [42] ( E -value≤1e−5). Homologous genome sequences were then aligned to the matching proteins that were identified as having synteny using Genewise [43] , to define gene models. For de novo prediction, Augustus [44] and Genscan [45] were used to predict coding genes. Finally, the homology-based and de novo -derived gene sets were merged using GLEAN ( http://sourceforge.net/projects/glean-gene/ ). For the Bactrian camel, LASTZ [46] was used to predict genes. Genes with coding lengths <150 bp were filtered out to reduce the number of false positives. Gene set evaluation and function annotation The CEGMA [7] pipeline, which contains 458 core eukaryotic genes that are highly conserved across a wide range of eukaryotes, was used to assess the completeness of the genomes and gene sets. The functions of genes were aligned based on the best match derived from the alignments to proteins annotated in the SwissProt, TrEMBL [47] , InterProscan [48] and Kyoto Encyclopedia of Genes and Genomes protein databases using Blastp. Repeat annotation and non-coding RNA annotation Tandem repeats were predicted using Tandem Repeats Finder [49] (version 4.04). Transposable elements (TEs) were identified in the genomes using a combination of homology-based and de novo approaches. For the homology-based approach, we first identified known TEs using RepeatMasker programme [50] against the Repbase [51] (version 16.10) database. We then used RepeatProteinMask [50] to identify TEs by aligning the genome sequence to the TE protein database. For the de novo method, we constructed a repeat library generated by RepeatModeler [52] , and RepeatMasker was used to identify the repeat sequences. The transfer RNA genes were predicted based on tRNAscan-SE [53] , and the ribosomal RNA fragments were identified by aligning human ribosomal RNA sequences to the camelid genomes using BLASTN. The micro RNA and small nuclear RNA genes were predicted by INFERNAL [54] software against the Rfam database [55] (Release 9.1) using the family-specific ‘gathering’ cutoff of Rfam. Gene family cluster and phylogenetic tree DNA and protein sequences for seven other mammals (human, mouse, cattle, horse, dog, panda and opossum) were downloaded from the Ensembl database (release 60). We used Treefam [56] methodology to define gene families. We constructed a phylogenetic tree based on 7,398 single-copy orthologous genes from these 10 species. Fourfold degenerate sites were extracted from each single family and concatenated to one supergene for each species. PHYML [57] was used to build phylogenetic trees under GTR+gamma for fourfold degenerate sites. Divergence time The coding sequences of 7,398 single-copy orthologous genes were used to estimate divergence times based on the phylogenetic tree. The PAML MCMCTREE [58] performs Bayesian estimation of species divergence times using soft fossil constraints [59] . The fossil calibration times were derived from a website ( http://www.fossilrecord.net ). Reconstruction of demographic history We used a PSMC model [14] with the generation time and mutation rates to reconstruct the most recent common ancestor distribution. We aligned short reads to the reference genome using BWA (version 0.5.9) [60] . The consensus sequences were obtained using SAMtools (version 0.1.17) [61] and divided into non-overlapping 100 bp bins. The resulting binned sequences were used as the input for the PSMC estimation. Positive selection We used PAML [58] to detect genes under positive selection. The branch-site model was used to identify positive genes for the two camels. We compared ModelA1, in which sites may evolve neutrally and under purifying selection, with ModelA, which allows sites to also be under positive selection. P -values were computed using the χ 2 -statistic adjusted by the false discovery rate method to allow for multiple testing. Rapidly evolving GO The approach based on Ka / Ks was used to identify GO categories that were significantly enriched or depleted in the object species. PRANK [62] was used to perform multiple sequence alignment of the single copies, and the lower-quality alignments were filtered using Gblocks [63] . The Ka and Ks values were then estimated using PAML. For a given GO category with more than 20 orthologues, the probability of observing an equal or higher number of non-synonymous substitutions was calculated assuming a binominal distribution. To determine whether a subset of the categories are evolving under significantly high (low) constraints, we repeated this procedure 10,000 times on the same data set after randomly permuting the GO annotations to test whether the probability was less than a threshold value. Finally, we selected the GO categories with P -values ≤0.01 for further analysis. Transcriptome sequencing and analysis All RNA samples were isolated from the renal cortex and medulla of eight female Bactrian camels. Four were randomly chosen as the CG, and the others were assigned to the WR. The Bactrian camels were fed hay with no water content ad libitum . The Bactrian camels in the WR group were not given water for 24 days, while the CG Bactrian camels drank water freely. Total RNA derived from the same treatment and same tissue were equally mixed to produce a single pool. After total RNA extraction, libraries were generated and sequenced using an Illumina HiSeq 2000 platform. Gene expression levels were measured by reads per kilobase per million mapped reads [64] . Differentially expressed genes (DEGs) were detected according to a method [65] . All DEGs were mapped to GO terms in the database ( http://www.geneontology.org/ ) and the number of genes for every term were calculated to identify GO terms that were significantly enriched in the input list of DEGs. Accession codes: The Camelid Whole Genome Shotgun Project has been deposited in DDBJ/EMBL/GenBank under accession codes JARL00000000 (Bactrian camel), JDVD00000000 (dromedary) and JEMW00000000 (alpaca). Raw DNA sequencing reads have been submitted to the NCBI Sequence Read Archive database under accession codes SRA179184 (Bactrian camel), SRA179175 (dromedary) and SRA179183 (alpaca). How to cite this article: Wu, H. et al . Camelid genomes reveal evolution and adaptation to desert environments. Nat. Commun. 5:5188 doi: 10.1038/ncomms6188 (2014).